Interplay between trigger factor and other protein biogenesis factors on the ribosome Nascent proteins emerging from translating ribosomes in bacteria are screened by a number of ribosome-associated protein biogenesis factors, among them the chaperone trigger factor (TF), the signal recognition particle (SRP) that targets ribosomes synthesizing membrane proteins to the membrane and the modifying enzymes, peptide deformylase (PDF) and methionine aminopeptidase (MAP). Here, we examine the interplay between these factors both kinetically and at equilibrium. TF rapidly scans the ribosomes until it is stabilized on ribosomes presenting TF-specific nascent chains. SRP binding to those complexes is strongly impaired. Thus, TF in effect prevents SRP binding to the majority of ribosomes, except those presenting SRP-specific signal sequences, explaining how the small amount of SRP in the cell can be effective in membrane targeting. PDF and MAP do not interfere with TF or SRP binding to translating ribosomes, indicating that nascent-chain processing can take place before or in parallel with TF or SRP binding. During protein biosynthesis, the nascent peptide chains on translating ribosomes are scanned by a number of protein ligands, called ribosome-associated protein biogenesis factors (RPBs), such as the chaperone trigger factor (TF), the signal recognition particle (SRP) and the processing enzymes peptide deformylase (PDF) and methionine aminopeptidase (MAP). RPBs bind to the ribosome close to the exit of the emerging nascent peptide by attaching to a confined binding platform comprising six ribosomal proteins surrounding the polypeptide tunnel exit ( Fig. 1 ). Whether co-translational binding of these ligands is regulated and to which extent RPBs can bind simultaneously or compete for binding is not clear [1] . 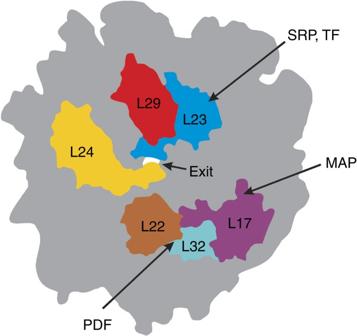Figure 1: Binding platform for RPBs at the peptide exit of the bacterial 50S ribosomal subunit. Ribosomal proteins at or near the peptide exit of the 50S subunit (grey outline) are indicated along with the RPBs binding to protein L23 (SRP, TF), L22 (PDF) or L17 (MAP) (for references, see text). Figure 1: Binding platform for RPBs at the peptide exit of the bacterial 50S ribosomal subunit. Ribosomal proteins at or near the peptide exit of the 50S subunit (grey outline) are indicated along with the RPBs binding to protein L23 (SRP, TF), L22 (PDF) or L17 (MAP) (for references, see text). Full size image TF is an early-acting ribosome-associated chaperone that binds nascent proteins emerging from the ribosome and prevents co-translational misfolding of these proteins [2] , [3] , [4] . TF is present in the cell in excess over ribosomes and potentially interacts with many nascent proteins [4] , [5] , with a preference for hydrophobic stretches flanked by positively charged amino acids [6] . Structural and mechanistic aspects of TF function have been reviewed recently [4] , [7] , [8] . SRP initiates the targeting of ribosome nascent-chain complexes (RNCs) that are synthesizing membrane proteins to the protein-conducting channel (translocon) in the plasma membrane [9] , [10] , [11] . SRP scans translating ribosomes for emerging hydrophobic signal-anchor sequences (SAS). Binding to an SAS switches SRP to the targeting mode and initiates co-translational membrane targeting by binding to the SRP receptor and transfer to the translocon [12] , [13] . SRP and TF together can bind to the ribosome, although both contact protein L23 at the peptide exit ( Fig. 1 ) [3] , [14] , [15] , [16] , [17] , [18] ; changes in crosslinking patterns indicate that conformational changes accompany the accommodation of the two ligands on one ribosome [19] , [20] . Depending on the functional state of the ribosome, the interaction of SRP with ribosomes takes place in different time domains. In the ‘scanning’ mode, SRP binds to non-translating ribosomes or ribosomes that do not synthesize membrane proteins in a readily reversible fashion [13] , with effective dissociation rates in the range of 10 s −1 , allowing other RPBs to bind in a stochastic fashion. However, the extent to which RPBs can enter when SRP is stabilized on translating ribosomes with short nascent chains (‘stand-by’; effective off-rate about 1 s −1 ) or on ribosomes synthesizing membrane proteins (‘targeting’; effective off-rate about 0.1 s −1 ) [12] , [13] is not clear. The interplay of TF with other RPBs on the ribosome is not clear as well, as it has been reported that TF binds to and dissociates from ribosomes very slowly [21] , [22] , [23] , such that stably bound TF might interfere with the binding of other RPBs. Protein synthesis in bacteria starts with the incorporation of formylated methionine. Deformylation by PDF and removal of the N-terminal methionine by MAP are essential for the stability and function of many proteins [1] . The C-terminal helix of PDF has been located on the ribosome at protein L22 close to the peptide exit, suggesting how PDF might bind [24] . Current models argue that this location of PDF allows for early scanning and deformylation of nascent chains when they just appear outside the ribosomal exit tunnel. Deformylation and methionine removal occur on 60–80% of all proteins and control the stability of proteins, as the N-terminal amino acid determines the susceptibility of many mature proteins for the cellular protein degradation machinery [25] , [26] . It has been proposed that PDF and TF act in a concerted fashion [3] , whereas recent data from selective ribosome profiling indicated that TF and PDF do compete for ribosome binding in vivo [27] . Conversely, on the basis of binding data obtained in vitro , it was suggested that TF and SRP did not compete with PDF for binding to ribosomes or RNCs [28] . Although MAP binds to the ribosome at the peptide exit close to proteins L17 and L23, it does not compete with TF or SRP, but strongly competes with PDF [28] . To obtain quantitative data on the interplay of RPBs, including TF, SRP, PDF and MAP, at the peptide exit of the ribosome, we monitor fluorescence resonance energy transfer (FRET) between fluorophore-labelled ribosomes or RNCs and labelled TF or SRP. To relate competition binding data to the stability of the complexes, we measure the interaction of TF with non-translating ribosomes as well as with RNCs, including the kinetics of complex formation and dissociation. We observe that TF rapidly binds to, and dissociates from vacant or translating ribosomes, unless nascent chains comprising TF-specific binding sites are presented, which strongly stabilize the complex. The competition between TF and SRP and other RPBs for binding to the ribosome is examined at equilibrium providing quantitative data that reveal the choreography of RPBs at the ribosomal peptide exit. The data reveal that simultaneous binding of TF and SRP to one ribosome lowers the binding affinity about 10-fold. Thus, in effect, TF precludes SRP binding to TF-specific RNCs. In contrast, the binding of PDF or MAP to RNCs does not influence the binding of TF or SRP. Kinetics of TF interaction with non-translating ribosomes To determine the kinetics of TF–ribosome complexes, we monitored TF binding to, and dissociation from, ribosomes by FRET between ribosomes labelled with 7-Diethylamino-3-((((2-Maleimidyl)ethyl)amino)carbonyl)coumarin (MDCC; donor) at position 21 of protein L23 (ref. 13 ) and TF labelled with Bodipy-FL (Bpy; acceptor) at position 99. To examine the kinetics of ribosome–TF complex formation, we rapidly mixed MDCC-labelled ribosomes with TF(Bpy) and monitored the increase of the acceptor signal ( Fig. 2a ). The signal change was single exponential, and long-time measurements did not reveal any additional slow step ( Supplementary Fig. 1a ). To verify that the signal change observed on binding of labelled TF to ribosomes was due to FRET, we performed a control experiment with ribosomes containing cysteine-free wild-type L23, which had been reacted with MDCC, leading to low-level incorporation of MDCC at proteins other than L23. Essentially, no signal change was observed with those ribosomes ( Supplementary Fig. 1b ), confirming that the signal changes observed with L23-labelled ribosomes were due to FRET and reported complex formation between TF and ribosomes. 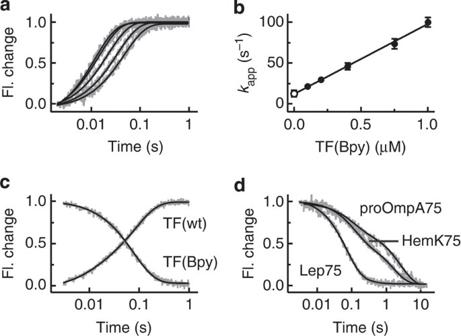Figure 2: Rapid kinetics of TF–ribosome interaction. (a) Complex formation. Binding of TF(Bpy) to MDCC-labelled ribosomes was monitored by Bpy fluorescence (Methods). TF(Bpy) concentrations (μM): 0.1, 0.2, 0.4, 0.75, 1.0, bottom to top. Time courses of the fluorescence change (Fl. change) are plotted; the concentration dependence was measured at least twice independently. Single-exponential fitting (continuous lines) yielded apparent rate constants (kapp) depicted inb. (b) Concentration dependence. Values ofkappfromaare plotted against the TF(Bpy) concentration (filled circles); the dissociation rate (open circle) was measured directly (cf.c) and included in the fit. Error bars are standard errors of the fits ina. (c) Complex dissociation. In the direct dissociation experiment, the dissociation of the preformed ribosome–TF(Bpy) complex, as induced by mixing with excess unlabelled TF, was monophasic,koff=12 s−1. In the indirect experiment, MDCC-labelled ribosomes with prebound unlabelled TF were rapidly mixed with TF(Bpy), and Bpy fluorescence was monitored. Double-exponential fitting yielded a rapid step (kapp1, 20% amplitude), due to direct binding of TF(Bpy) to a small amount of vacant ribosomes, and a slower step (kapp2=12 s−1, 80% amplitude) due to TF(Bpy) binding which was rate-limited by the dissociation of prebound TF. (d) Dissociation of TF from RNCs. The complexes of TF(Bpy) with MDCC-labelled RNCs were rapidly mixed with excess unlabelled TF. Time courses obtained with proOmpA75-RNC and HemK75-RNC were evaluated by two-exponential fitting. One time constant,kapp1, was due to the dissociation of TF from non-translating ribosomes, and another,kapp2, to TF dissociation from the respective RNC. The dissociation of TF(Bpy) from Lep75-RNCs was monophasic, and single-exponential fitting yieldedkapp1=koff=12 s−1, as for non-translating ribosomes. Figure 2: Rapid kinetics of TF–ribosome interaction. ( a ) Complex formation. Binding of TF(Bpy) to MDCC-labelled ribosomes was monitored by Bpy fluorescence (Methods). TF(Bpy) concentrations (μM): 0.1, 0.2, 0.4, 0.75, 1.0, bottom to top. Time courses of the fluorescence change (Fl. change) are plotted; the concentration dependence was measured at least twice independently. Single-exponential fitting (continuous lines) yielded apparent rate constants ( k app ) depicted in b . ( b ) Concentration dependence. Values of k app from a are plotted against the TF(Bpy) concentration (filled circles); the dissociation rate (open circle) was measured directly ( cf. c ) and included in the fit. Error bars are standard errors of the fits in a . ( c ) Complex dissociation. In the direct dissociation experiment, the dissociation of the preformed ribosome–TF(Bpy) complex, as induced by mixing with excess unlabelled TF, was monophasic, k off =12 s −1 . In the indirect experiment, MDCC-labelled ribosomes with prebound unlabelled TF were rapidly mixed with TF(Bpy), and Bpy fluorescence was monitored. Double-exponential fitting yielded a rapid step ( k app1 , 20% amplitude), due to direct binding of TF(Bpy) to a small amount of vacant ribosomes, and a slower step ( k app2 =12 s −1 , 80% amplitude) due to TF(Bpy) binding which was rate-limited by the dissociation of prebound TF. ( d ) Dissociation of TF from RNCs. The complexes of TF(Bpy) with MDCC-labelled RNCs were rapidly mixed with excess unlabelled TF. Time courses obtained with proOmpA75-RNC and HemK75-RNC were evaluated by two-exponential fitting. One time constant, k app1 , was due to the dissociation of TF from non-translating ribosomes, and another, k app2 , to TF dissociation from the respective RNC. The dissociation of TF(Bpy) from Lep75-RNCs was monophasic, and single-exponential fitting yielded k app1 = k off =12 s −1 , as for non-translating ribosomes. Full size image Time courses ( Fig. 2a ) were evaluated by single-exponential fitting and yielded apparent rate constants ( k app ) that increased with the TF(Bpy) concentration in a linear fashion ( Fig. 2b ), indicating a second-order binding step. The linear fit yielded the rate constants of complex formation and dissociation, k on and k off ( Table 1 ). The same value for k off we obtained directly by monitoring the dissociation of the ribosome–TF(Bpy) complex as induced by mixing with excess unlabelled TF ( Fig. 2c ). Unlabelled TF dissociated from the ribosome at the same rate, as shown by experiments in which the binding of TF(Bpy) to ribosomes was rate limited by the dissociation of prebound unlabelled TF ( Fig. 2c ). Thus, the Bpy label at position 99 did not influence the interaction of TF with ribosomes. The equilibrium dissociation constant ( K d ) of the TF complex with non-translating ribosomes, as calculated from the rate constants ( Table 1 ), was comparable to the value obtained by equilibrium titration ( Supplementary Fig. 2 ) and values reported previously [19] , [29] . Table 1 Parameters of TF binding to non-translating ribosomes and RNCs*. Full size table The kinetic analysis revealed that the TF–ribosome complex forms rapidly with an association rate constant around 100 μM −1 s −1 , which is close to the limit set by diffusion. Furthermore, the TF complex with non-translating ribosomes in our analysis is unstable, with a short half-life time of about 60 ms ( k off =12 s −1 ). These results are at variance with previous studies on the kinetics of TF–ribosome interaction, obtained by monitoring the fluorescence of a BADAN label at position 14 of TF, which reported very low rates of complex formation and dissociation [21] , [22] , [23] . As described in the Supplementary Note , we have repeated the analysis with BADAN-labelled TF and observed similarly low rates ( Supplementary Fig. 3 ). One possible explanation for the slow kinetics could be a slow rearrangement between non-binding and binding conformations of TF ( Supplementary Fig. 3c ) that is characteristic for BADAN-labelled TF and is not observed with TF(Bpy) labelled at position 99. TF interaction with RNCs To study the influence of nascent chains with or without TF-specific sequences on the interaction of TF with RNCs, we have used MDCC-labelled RNCs carrying various nascent chains. The length of the nascent chain was restricted to 75 amino acids to avoid TF binding to longer nascent chains off the ribosome [5] . The affinities of TF for binding to those RNCs we determined by equilibrium titrations ( Supplementary Fig. 2 ; Table 1 ). TF bound very strongly ( K d =2.5 nM) when translating ribosomes displayed the nascent chain of proOmpA, which contains a TF-binding motif consisting of an extended hydrophobic patch with flanking positive charges [6] . Furthermore, TF bound to HemK75-RNCs rather strongly, consistent with the presence of a similar TF-binding motif in nascent HemK. In contrast, Lep75-RNCs bound TF with low affinity as vacant ribosomes, indicating that TF does not interact with the hydrophobic signal-anchor sequence of Lep. However, given the high concentration of TF in the cell (about 50 μM total [30] ), TF can probably bind to most ribosomes, including non-translating ribosomes and RNCs, even to those RNCs that do not present a TF-binding motif. This raises the question of how the other RPBs gain access to the nascent peptide for N-terminal processing (PDF, MAP) and membrane targeting (SRP). One possibility would be rapid dissociation of TF, allowing alternate binding of RPBs at sufficient speed, another concurrent binding of TF and the other RPBs. These possibilities are examined in the following. To assess the kinetic stabilities of different TF–RNC complexes, we rapidly mixed the complexes containing TF(Bpy) with a large excess of unlabelled TF ( Fig. 2d ). With proOmpA75- and HemK75-RNC, the observed time courses were biphasic with a rapid phase reflecting the dissociation of TF from non-translating ribosomes, which were present in the RNC preparations at a level of about 10% (but contributed nearly half of the total amplitude, due to the large FRET change accompanying the formation or dissociation of the TF complex with non-translating ribosomes, compared with proOmpA-RNC; cf . Fig. 3a,c ). The slow phase was only observed with RNCs that strongly bind TF and was, therefore, attributed to the dissociation of the respective TF–RNC complex. According to this analysis, the complex of TF with proOmpA75-RNCs is stabilized strongly ( k off ≈0.4 s −1 ), compared with the complex with non-translating ribosomes, in accordance with the equilibrium data ( Table 1 ). A similar stabilization we observed with HemK75-RNC. The dissociation of TF from Lep75-RNC gave rise to a single-exponential time course ( k off ≈12 s −1 ), as with non-translating ribosomes, indicating that an interaction of TF with the nascent Lep peptide, although it comprises a hydrophobic element, does not contribute significantly to the stability of the complex, again in accordance with the equilibrium titration. Comparable observations have been made previously with RNCs comprising various hydrophobic sequence elements, although half-life times of RNC–TF complexes generally were much longer [5] . 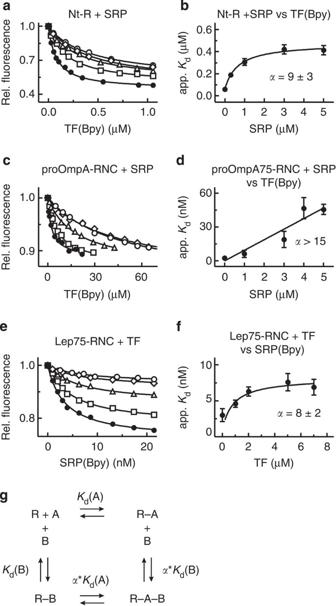Figure 3: Partial competitive binding of TF and SRP to ribosomes and RNCs. (a) Effect of SRP on TF(Bpy) binding to non-translating ribosomes. ApparentKdvalues were obtained by fitting a quadratic equation for ligand binding to one site. SRP concentrations (μM): None, •; 0.3, □; 1.0, Δ; 3.0,; 5.0,○. (b) ApparentKdvalues. Error bars represent the standard error of the fits. The data were evaluated by fitting an equation for partial competitive binding derived for the model depicted ing, to yield the indicatedαfactor with the standard error of the fit (Methods). (c) TF(Bpy) binding to proOmpA75-RNC. SRP concentrations (μM): None, •; 1.0, □; 3.0, Δ; 4.0,; 5.0,○. (d) Plot of apparentKdvalues fromcagainst SRP concentration. Only a lower limit forαwas obtained, because due to very weak binding saturation with SRP could not be reached. (e) SRP(Bpy) binding to Lep75-RNC in the presence of increasing concentrations of TF (μM): None, •; 1.0, □; 2.0, Δ; 5.0,; 7.0,○. (f) ApparentKdvalues frome. Non-linear fitting as inayielded theαfactor. (g) Model of partial competitive binding. The model describes concurrent ribosome (R) binding of ligands A and B, defining a factorαby which the apparentKdof ligand A is increased over the initial, intrinsicKdat saturation with ligand B, and vice versa. Figure 3: Partial competitive binding of TF and SRP to ribosomes and RNCs. ( a ) Effect of SRP on TF(Bpy) binding to non-translating ribosomes. Apparent K d values were obtained by fitting a quadratic equation for ligand binding to one site. SRP concentrations (μM): None, •; 0.3, □; 1.0, Δ; 3.0, ; 5.0, ○ . ( b ) Apparent K d values. Error bars represent the standard error of the fits. The data were evaluated by fitting an equation for partial competitive binding derived for the model depicted in g , to yield the indicated α factor with the standard error of the fit (Methods). ( c ) TF(Bpy) binding to proOmpA75-RNC. SRP concentrations (μM): None, •; 1.0, □; 3.0, Δ; 4.0, ; 5.0, ○ . ( d ) Plot of apparent K d values from c against SRP concentration. Only a lower limit for α was obtained, because due to very weak binding saturation with SRP could not be reached. ( e ) SRP(Bpy) binding to Lep75-RNC in the presence of increasing concentrations of TF (μM): None, •; 1.0, □; 2.0, Δ; 5.0, ; 7.0, ○ . ( f ) Apparent K d values from e . Non-linear fitting as in a yielded the α factor. ( g ) Model of partial competitive binding. The model describes concurrent ribosome (R) binding of ligands A and B, defining a factor α by which the apparent K d of ligand A is increased over the initial, intrinsic K d at saturation with ligand B, and vice versa. Full size image To obtain rate constants for the association of TF with ribosomes or RNCs, we monitored the FRET change on rapidly mixing MDCC-labelled RNCs with TF(Bpy). One- or two-exponential fitting of the time courses yielded apparent rate constants for TF binding to the small amount of non-translating ribosomes ( k app1 ), as above, and to the respective RNC ( k app2 ). The plots of the k app2 values against TF(Bpy) concentration ( Supplementary Fig. 4 ) were linear and did not level off at high concentration, indicating a one-step binding mechanism. Linear fitting of the plots gave the rate constants of TF–RNC complex formation and dissociation, k on and k off ( Table 1 ); similar k off values were directly determined by chase ( Fig. 2d ). The association rate constants for non-translating ribosomes and the RNCs differed by less than threefold, indicating that the presence of nascent chains did not appreciably affect the association of TF. Thus, the higher affinity of TF binding to RNCs presenting TF-binding motifs (HemK, proOmpA) was predominantly due to lower dissociation rates. Interplay between TF and SRP on the ribosome According to previous qualitative data, TF and SRP can bind simultaneously to vacant ribosomes and RNCs, and concurrent binding is accompanied by rearrangements of the complex [19] , [20] . To examine concurrent binding of TF and SRP quantitatively, we performed equilibrium titrations in which the binding of TF(Bpy) or SRP(Bpy) to MDCC-labelled non-translating ribosomes or RNCs was measured in the presence of increasing amounts of the respective other ligand ( Fig. 3 ). Titration curves were evaluated by fitting using a quadratic equation (Methods), yielding K d values and the maximum FRET difference at saturation. Changes of FRET levels at saturation with TF(Bpy) indicate structural rearrangements of the ribosome–TF(Bpy) complex induced by SRP binding, rather than TF(Bpy) displacement. The final fluorescence levels without or with added SRP were similar with non-translating ribosomes (40 and 55% fluorescence decrease; Fig. 3a ) or proOmpA75-RNC (10 to 15% fluorescence decrease; Fig. 3c ), indicating that the SRP-induced conformational changes of the TF complexes were not large. Nevertheless, SRP-induced conformational readjustments of ribosome–TF complexes may affect the binding affinity. In fact, SRP binding decreased the affinity of TF binding to non-translating ribosomes ( Fig. 3a,b ) or proOmpA75-RNC ( Fig. 3c,d ). To quantify the effect, the titration data were evaluated in terms of a general binding model that allowed for concurrent binding of TF and SRP and accounted for apparent affinity changes by introducing a factor α , describing the affinity decrease in the presence of the competitor ( Fig. 3g ; Methods). According to this analysis, concurrent binding of SRP decreased the affinity of TF binding to non-translating ribosomes by a factor α =9 ( Fig. 3b ). The evaluation also yielded the intrinsic dissociation constants for SRP, about 80 nM, and TF, about 100 nM, both in accordance with the values obtained by direct titration (ref. 12 ; Supplementary Fig. 2 ), underscoring the validity of the model. The effect of SRP on TF binding to proOmpA75-RNCs appeared similar, although the very low binding affinity of SRP ( K d =0.8 μM; Supplementary Fig. 2 ) precluded that saturation with SRP was reached; thus, only a lower limit for the α factor, about 15, could be determined ( Fig. 3d ). Furthermore, an α factor of 8 was determined for the effect of TF on the binding of SRP to Lep75-RNC ( Fig. 3e,f ). Thus, we conclude that concurrent binding of TF and SRP to non-translating ribosomes or RNCs exposing TF or SRP-specific nascent peptides weakens the binding of either RPB about 10-fold. Effect of PDF on ribosome binding of TF and SRP Next, we addressed the question whether PDF influences the binding of TF or SRP to ribosomes, and vice versa. The presence of PDF substantially reduced the FRET change accompanying TF binding to non-translating ribosomes, which decreased by only 5% in the presence of saturating amounts of PDF, compared with 55% in the absence of PDF ( Fig. 4a ). This indicated that TF remained bound when PDF was bound to the ribosome, but in a changed arrangement. The results obtained with PDF, SRP and non-translating ribosomes were similar ( Fig. 4c ), in that the change of FRET accompanying the titrations became smaller with increasing PDF concentration (from 40 to 20% decrease). The evaluation of the titrations on the basis of the partial competition model of Fig. 3g yielded respective α factors of about 15 or 5 for the effect of PDF on the affinities of TF or SRP binding to non-translating ribosomes ( Fig. 4b,d ). Furthermore, the fitting yielded intrinsic K d values for the binding of TF, around 50 nM, and SRP, around 80 nM, consistent with the values obtained by direct titration in the absence of competitor ( Supplementary Fig. 2 ; Bornemann et al . [12] ). Finally, the evaluation of the titrations yielded an intrinsic K d of PDF binding to non-translating ribosomes of around 1.5 μM, comparable to a published value [28] . 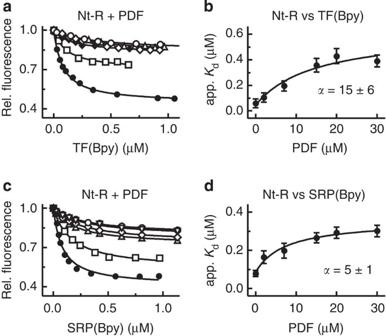Figure 4: Partial competitive binding of PDF and TF or SRP to non-translating ribosomes. (a) TF(Bpy) binding to ribosomes in the presence of increasing concentrations of PDF. Complex formation was measured as inFig. 3at increasing concentrations of PDF (μM): None, •; 2.0, □; 7.0, Δ; 15,; 20,○; 30,∇. (b) Plot of apparentKdvalues fromaagainst PDF concentration. Errors were estimated as inFig. 3. The plot was evaluated by fitting as inFig. 3to yield theαfactor as indicated. (c) SRP(Bpy) binding to ribosomes in the presence of increasing concentrations of PDF. Concentrations of PDF were as ina. (d) Plot of the apparentKdvalues fromcagainst PDF concentration. Figure 4: Partial competitive binding of PDF and TF or SRP to non-translating ribosomes. ( a ) TF(Bpy) binding to ribosomes in the presence of increasing concentrations of PDF. Complex formation was measured as in Fig. 3 at increasing concentrations of PDF (μM): None, •; 2.0, □; 7.0, Δ; 15, ; 20, ○ ; 30, ∇ . ( b ) Plot of apparent K d values from a against PDF concentration. Errors were estimated as in Fig. 3 . The plot was evaluated by fitting as in Fig. 3 to yield the α factor as indicated. ( c ) SRP(Bpy) binding to ribosomes in the presence of increasing concentrations of PDF. Concentrations of PDF were as in a . ( d ) Plot of the apparent K d values from c against PDF concentration. Full size image The effects of PDF on TF or SRP binding to their respective cognate RNCs were different. In both cases, the addition of increasing amounts of PDF resulted in the gradual loss of fluorescence amplitudes (initially about 10% decrease), such that at saturating PDF concentration the complex formation was not detectable ( Fig. 5a,b ). However, the titrations in which the binding of TF(Bpy) or SRP(Bpy) was still observable (up to 1 or 2 μM PDF) showed that the affinities for the binding of TF(Bpy) or SRP(Bpy) were not changed significantly ( Fig. 5c ). Thus, the competition model introduced above, which implies changes of K d , does not apply for PDF on RNCs. The simplest model consistent with the results would be that PDF can bind concurrently with TF or SRP and does not influence their binding affinities. However, PDF binding has some influence on the arrangement of TF and SRP on their respective substrate RNCs, as indicated by the loss of FRET with increasing concentrations of PDF. 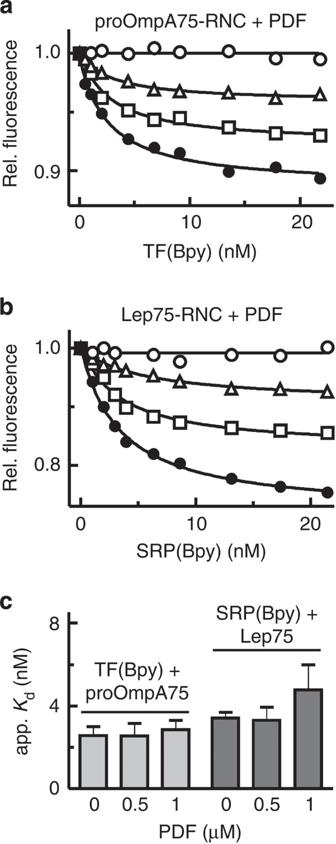Figure 5: Non-competitive binding of PDF and TF(Bpy) or SRP(Bpy) to RNCs. (a) TF(Bpy) binding to proOmpA75-RNCs in the presence of increasing amounts of PDF. Complex formation was monitored in the presence of PDF (μM): None, •; 0.5, □; 1.0, Δ; 5.0,○. (b) SRP(Bpy) binding to Lep75-RNCs in the presence of increasing amounts of PDF. Complex formation was monitored as ina. (c)Kdvalues fromaandbdetermined at the indicated PDF concentrations. Errors were estimated as inFig. 3. Figure 5: Non-competitive binding of PDF and TF(Bpy) or SRP(Bpy) to RNCs. ( a ) TF(Bpy) binding to proOmpA75-RNCs in the presence of increasing amounts of PDF. Complex formation was monitored in the presence of PDF (μM): None, •; 0.5, □; 1.0, Δ; 5.0, ○ . ( b ) SRP(Bpy) binding to Lep75-RNCs in the presence of increasing amounts of PDF. Complex formation was monitored as in a . ( c ) K d values from a and b determined at the indicated PDF concentrations. Errors were estimated as in Fig. 3 . Full size image Small effect of MAP on ribosome binding of TF and SRP It is not known to which extent the binding of MAP, which may enter RNCs early during protein synthesis, influences the binding of TF or SRP. On addition of MAP in saturating concentrations, K d values for TF or SRP increased less than twofold for the complexes with non-translating ribosomes or the respective RNCs ( Supplementary Fig. 5 ). Fluorescence amplitude changes were small as well. These results indicate that MAP bound to ribosomes, as reported recently [28] , and did not displace TF or SRP from non-translating ribosomes or RNCs or change affinities. One major finding of this paper is that TF rapidly forms transient complexes with ribosomes. The kinetic stability of the complexes depends on the functional state of the ribosomes and the nature of the nascent peptide presented on the ribosome. Ribosome–TF complexes form with second-order rate constants of 100–200 μM −1 s −1 , that is, complex formation is close to diffusion controlled. The complexes are short-lived, with half-life times of 60 ms, when the ribosomes are vacant or present a nascent protein lacking a TF-binding motif, such as in Lep75-RNC; in these cases binding affinities are in the range of 0.1–0.2 μM. The ribosome–TF complexes are strongly stabilized (20–30-fold) and binding affinities are high ( K d values of 2–10 nM) when RNCs expose nascent peptides encompassing TF-binding sequences, such as in the proOmpA75- or HemK75-RNCs used here. Up to about 20-fold higher K d values of TF binding to vacant ribosomes or various RNCs, including RNCs presenting the nascent beta subunit of RNA polymerase, a TF substrate, were reported previously [31] . However, those values were obtained by pelleting ribosome–TF complexes, which apparently underestimated affinities, in particular when the complexes were unstable kinetically, such as the complexes with vacant ribosomes or Lep-RNCs. The present parameters of TF–ribosome interaction also differ from published values determined using fluorescence-labelled TF [21] , [22] , [23] . In that work, half-life times around 10 s and equilibrium dissociation constants of 1–2 μM were observed for the complexes of labelled TF with non-translating ribosomes and half-life times up to 50 s for translating ribosomes exposing TF-binding nascent chains [21] , [22] , [23] . However, as we show here, the slow kinetics of complex formation and dissociation as well as low-affinity binding observed in those experiments were caused by the particular fluorescence label, BADAN at position 14, in TF that strongly influenced the properties of TF. A transient character of ribosome–TF complexes resolves the potential problem of slowly forming and long-lived TF complexes with translating ribosomes, including non-substrate RNCs, which might interfere with nascent-chain processing by PDF and MAP and/or membrane targeting by SRP, despite concurrent binding. Thus, rather than staying bound on translating ribosomes and ‘waiting’ for nascent peptides to emerge from the exit tunnel, as suggested by the previously reported slow kinetics, the interaction of TF with ribosomes appears highly dynamic. An off-rate of about 12 s −1 matches a translation rate of 10 s −1 and, combined with a high effective on-rate (≈1,000 s −1 , based on an approximate second-order association rate constant of ≈100 μM −1 s −1 and assuming ≈10 μM free TF monomer in the monomer–dimer equilibrium [32] ) allows TF to inspect many translating ribosomes at appropriate speed and settle on TF-specific sequences as soon as they emerge from the exit tunnel. This may be important for the chaperone function of TF in preventing premature, potentially erroneous folding of nascent proteins. Previous kinetic analyses revealed that, similar to what we report here for TF, SRP scans ribosomes rapidly until binding is stabilized on translating ribosomes that have their peptide exit tunnel filled (‘stand-by’) or expose a signal-anchor sequence (‘targeting’) [13] . Assuming an SRP concentration in vivo of 0.1 μM and diffusion-controlled binding, as observed in vitro [13] , the effective rate of SRP binding to ribosomes or RNCs is about 10 s −1 . This rate matches the rate of TF dissociation from non-TF-substrate RNCs, Lep75-RNC in our experiments, which may optimize the access of SRP to its substrate RNCs. The observed destabilization of SRP binding to non-substrate RNCs by high-affinity TF binding to TF-substrate RNCs enhances the specificity, in particular of SRP, for binding to its substrate RNCs ( Fig. 6 ). Although SRP and TF can bind to ribosomes concurrently, the destabilization has the consequence that SRP is practically excluded from the large number of RNCs to which TF is bound strongly [5] . Rather, SRP will predominantly be bound to RNCs with short nascent peptides filling the exit tunnel and, in particular, RNCs presenting an SAS, as SRP binds to those RNCs with an apparent K d ≈20 nM even at saturation with TF, which is well below the intracellular concentration of SRP of around 100 nM. Thus, the partial competitive binding behaviour of TF and SRP in effect increases the specificity of the small amount of SRP present in the cell in promoting co-translational membrane targeting of those RNCs that synthesize membrane proteins. 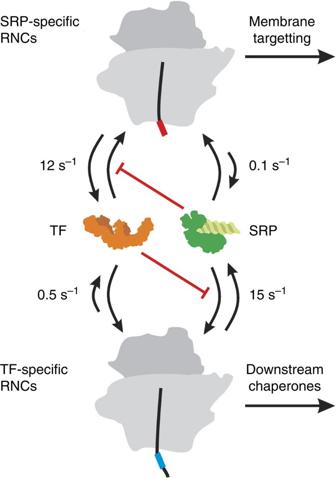Figure 6: Interplay of TF and SRP on translating ribosomes. Concurrent binding of TF or SRP to RNCs presenting the respective specific nascent chain (SRP-specific SAS, red; TF-specific sequence, blue) leads to weakening of the binding of the respective other ligand (values ofKdincreased eightfold or >15-fold, respectively (Fig. 3)), as indicated by red lines. Because SRP dissociates from RNCs in three steps, average values ofkoffcalculated from the three rate constantsk−1,k−2andk−3are given13. Values ofkofffor TF dissociation from RNCs are taken fromTable 1. Second-order rate constants for TF or SRP binding to RNCs ranged from about 100 to 200 μM−1s−1(Table 1and ref.13), indicating near diffusion-controlled binding. Figure 6: Interplay of TF and SRP on translating ribosomes. Concurrent binding of TF or SRP to RNCs presenting the respective specific nascent chain (SRP-specific SAS, red; TF-specific sequence, blue) leads to weakening of the binding of the respective other ligand (values of K d increased eightfold or >15-fold, respectively ( Fig. 3 )), as indicated by red lines. Because SRP dissociates from RNCs in three steps, average values of k off calculated from the three rate constants k −1 , k −2 and k −3 are given [13] . Values of k off for TF dissociation from RNCs are taken from Table 1 . Second-order rate constants for TF or SRP binding to RNCs ranged from about 100 to 200 μM −1 s −1 ( Table 1 and ref. 13 ), indicating near diffusion-controlled binding. Full size image The binding of PDF to TF complexes with non-translating ribosomes results in weakening of those complexes, as the apparent K d of TF binding was 15-fold higher than the intrinsic K d , indicating partial competitive binding. The SRP complexes with non-translating ribosomes behave similarly, in that concurrent binding of PDF is accompanied by rearrangements and a fivefold increase of the apparent K d of SRP binding. Qualitative data indicated concurrent binding of TF and PDF or SRP and PDF to non-translating ribosomes or RNCs exposing the signal sequence of DsbA, a secretory protein that is recognized by SRP and translocated to the periplasm co-translationally [28] . These results are supported by the present quantitative analysis, in that the binding of PDF to either proOmpA75-RNC or Lep75-RNC has no influence on the binding affinity of TF or SRP, respectively, indicating non-competitive binding. Parallel binding combined with rapid scanning of TF is consistent with the binding preferences of PDF and TF. Whereas PDF can act on ribosomes exposing short nascent chains independent of the sequence [1] , or even on isolated short oligopeptides, TF binding to RNCs with short nascent chains is transient, and the complex is stabilized when nascent chains containing TF-specific hydrophobic patches become available. Thus, PDF and TF can act sequentially, in accordance with the observed rapid kinetics of PDF binding to ribosomes [28] and the binding preference of TF for RNCs carrying nascent peptides of about 100 amino acids or longer observed by directed ribosome profiling in vivo [27] . In contrast, SRP is recruited to translating ribosomes early, even before the nascent peptide emerges from the exit tunnel [12] , and forms a rather stable complex (half-life time about 0.5 s, ref. 13 ). Thus, SRP with high probability will remain bound to the ribosome until continued translation exposes a hydrophobic TM segment, which further stabilizes the complex (half-life time about 5 s) and initiates targeting of the RNC to the translocon. (When sequences of non-membrane proteins emerge from the ribosome, the complexes are destabilized ( Supplementary Fig. 2e ; ref. 12 ) and SRP is released rapidly [13] ) Regarding PDF, our data show that it can bind concurrently to RNC–TF or RNC–SRP complexes without appreciable effects on these complexes, and there are indications that PDF deformylates the N terminus of the nascent peptide before the binding of TF [28] . It remains to be examined, however, whether PDF can access and deformylate the N terminus of the nascent peptide when it is bound to SRP. Materials 4.5S RNA and mRNAs coding for the first 75 amino acids of leader peptidase (Lep), HemK, or proOmpA were prepared by in vitro transcription of linearized DNA generated from plasmid pT7-4.5S for 4.5S RNA and plasmid pBSK2-LepB for Lep75 mRNA, using Phusion polymerase (Biozym). The mRNAs for proOmpA75 and HemK75 were prepared in the same way, using pUC19-derived plasmids as templates. Ffh, PDF and MAP, all extended by six histidines at the C terminus, were expressed in E. coli BL21(DE3)pLysS from pET24-derived plasmids. Ffh was purified by affinity chromatography (Ni-NTA) followed by ion exchange chromatography (SP Sepharose) [33] . PDF was purified by Talon affinity metal agarose (Clontech) followed by Q-Sepharose in the presence of 5 mM CoCl 2 (ref. 34 ). MAP was purified by affinity chromatography (Ni-NTA). Remaing impurities were removed by size exclusion chromatography (Superdex 75) [35] . TF was expressed from plasmid pCA528 and purified in two steps. The SUMO-tagged protein was first purified by Ni-NTA chromatography. Subsequently, the SUMO-tag was cleaved off by incubation with His-tagged ULP-1 protease for 2h. The protease was then removed by binding to Ni-NTA [36] . Proteins were stored at −80°C in buffer A (25 mM HEPES, pH 7.5, 70 mM NH 4 Cl, 30 mM KCl, 7 mM MgCl 2 , 0.2 mM CoCl 2 , 10% glycerol). The addition of 0.2 mM CoCl 2 was necessary and sufficient to keep both PDF and MAP active [37] , [38] ; higher concentrations of CoCl 2 slowed down the rate of TF binding to ribosomes considerably. Fluorescence labelling QuickChange PCR mutagenesis using Phusion polymerase was performed to insert cysteine at position 430 of Ffh and positions 14 or 99 of TF. Mutations were confirmed by DNA sequencing. Mutant proteins were expressed and purified in the same way as the wild-type proteins. Labelling of cysteine-substituted Ffh and TF with the maleimide derivatives of the respective dye (Life Technologies) was carried out by incubation with a fivefold excess of dye over protein overnight at 4 °C [13] . The extent of labelling was 80–90%, based on absorption measurements and SDS polyacrylamide gel electrophoresis. For MDCC labelling of position 21 of protein L23, 50S ribosomal subunits were prepared from an L23-deficient E. coli strain (MC4100 ΔL23) harbouring the plasmid pTBL23S21C, which codes for the mutant protein L23(S21C). The purified 50S(L23S21C) subunits were then labelled by incubation with a 10-fold excess of MDCC-maleimide for 1 h at room temperature. Labelled 50S(L23S21C) subunits were associated with unlabelled 30S subunits to form active MDCC-labelled 70S ribosomes [13] . RNC preparation Ribosomes from E. coli MRE600, initiation factors IF1, IF2 and IF3, EF-Tu, EF-G, f[ 3 H]Met-tRNA fMet and total tRNA were prepared following standard procedures [39] . RNCs were prepared by in vitro translation of truncated mRNAs and purified by sucrose gradient centrifugation [12] . About 90% of the ribosomes carried the respective peptide chain. Lep35-RNC carrying a Bpy label at the N-terminal methionine of the nascent chain was prepared in the same way, except that Bpy-Met-tRNA fMet (ref. 40 ) was used for initiation complex formation. Rapid kinetics Rapid kinetic experiments were conducted by stopped flow in buffer A at 25°C, using a SX-20MV stopped-flow spectrometer (Applied Photophysics). Association kinetics of TF binding to ribosomes were measured by monitoring the fluorescence change after rapidly mixing equal volumes (55 μl) of the solution of MDCC-labelled ribosomes or RNCs (0.025 μM final concentration after mixing) with Bpy-labelled TF. The donor fluorophore, MDCC, was excited at 430 nm and the increase of acceptor (Bpy) emission was measured after passing a cut-off filter (KV530, Schott). To measure dissociation rates, complexes were prepared by incubating MDCC-labelled non-translating ribosomes (0.025 μM) or RNCs (0.015 μM) with TF(Bpy) (0.5 μM or 0.02 μM, respectively) for 5 min. To induce dissociation, the complexes were rapidly mixed with unlabelled TF (5 μM), and the decrease of Bpy fluorescence was monitored. The dissociation of unlabelled TF was measured analogously, starting with prebound unlabelled TF and monitoring the binding of TF(Bpy) added in excess, which was rate-limited by the dissociation of unlabelled TF. Stopped-flow time courses were evaluated by single- or double-exponential fitting, as indicated. Fluorescence titrations Titrations were performed in a Fluorolog 3 fluorimeter (Horiba) at 25 °C. The binding of TF(Bpy) or SRP(Bpy) to MDCC-labelled ribosomes was measured by FRET, monitoring the decrease of MDCC donor fluorescence. The excitation wavelength was 430 nm, and the emission was measured at 470 nm. Binding curves were evaluated by non-linear fitting, using a quadratic equation for ligand binding to one site. All titrations were performed at least two times and mean values are shown in the figures. Evaluation of partial competitive binding Competitive or partial competitive binding results in decreased affinities or an increase of the apparent K d . To quantify these effects, apparent K d values were determined by titrations with competing RPB. The plots of apparent K d versus concentration of competing RPB ( Figs 3 and 4 ) were evaluated by fitting to the following equation for partial competitive binding, derived for the model depicted in Fig. 3g : [B] denoting the concentration of competitor, K d (A) and K d (B) the intrinsic affinities of ligand A (for instance TF(Bpy or SRP(Bpy)) or B (the competitor). The observed apparent K d (A) at saturation with competitor differs from the intrinsic K d by a factor α . According to the model for partial competitive binding ( Fig. 3g ), the apparent K d of the competing ligand B is increased by the same factor. Fits are shown in Figs 3 and 4 along with the respective α factors. How to cite this article: Bornemann, T. et al. Interplay between trigger factor and other protein biogenesis factors on the ribosome. Nat. Commun. 5:4180 doi: 10.1038/ncomms5180 (2014).